Reply to: Accurate population proxies do not exist between 11.7 and 15 ka in North America 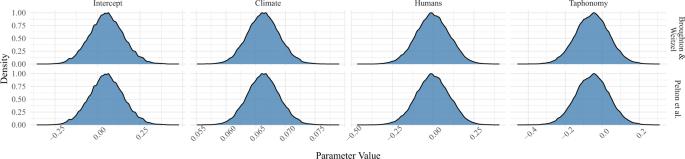Fig. 1: Regression results using vetted archaeological datasets. The effect of climate change, human population size, and taphonomy on megafauna population size using the vetted dates sets of Broughton and Weitzel3(top) and Pelton et al.4(bottom). Note that in both analyses the human posterior estimates overlap zero indicating indicates no relationship between human population size and megafauna population size. On the other hand, the posterior estimates for the climate change parameter do not overlap zero in either analysis indicating a significant effect. 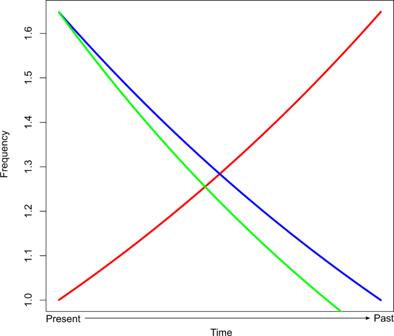Fig. 2: Possible effect of different taphonomic decay functions on change point position. Presented here are two hypothetical taphonomic decay functions (green, blue) and a hypothetical fossil count time-series (red). As shown, a slight shift in the rate of taphonomic decay causes a shift in the time at which it intersects with the fossil curve. Consequently, this will shift the timing of the change point and, given significant uncertainties in radiocarbon dating, may have significant ramifications for identifying coincidences between the appearance of Clovis culture and megafauna declines. The data Three key datasets were used in the present study. The first was compiled by Broughton and Weitzel [3] and comprised 521 radiocarbon-dated megafauna remains from the US and Canada. In our original study [1] we conducted some additional cleaning of the megafauna dataset to remove instances where multiple dates might derive from a single individual, as well as dates derived from plant remains. The resulting dataset comprised 432 radiocarbon-dated megafauna remains and was used in the present study. The second dataset was also compiled by Broughton and Weitzel and comprised 938 dates from archaeological contexts obtained from the Canadian Archaeological Radiocarbon Database (CARD). Pelton and colleagues flagged some of the dates as being potentially non-archaeological (see above). Following their recommendations, we cleaned the dataset to remove potentially non-archaeological dates for the present study. The final dataset used was the ~50-year resolved North Greenland Ice Core Project (NGRIP) δ 18 O record. For a full description of the methods and data used in the study we refer readers to Stewart et al. [1] . Radiocarbon-dated event count model For the extended analyses described above, we used the same Radiocarbon-dated Event Count (REC) model approach described in our original article [1] . These are Poisson regression models in which radiocarbon-dated samples comprise count sequences that are then compared to one or more covariates. As described in detail elsewhere [10] , radiocarbon dates contain substantial chronological uncertainty that has to be accounted for in quantitative analyses. REC models attempt to do so by employing a Bayesian hierarchical framework in which probable count sequences produced by randomly sampling individual radiocarbon dates in accordance with their distributions and then binning the dates into a temporal grid. These probable count sequences are treated like samples from a parent population that can be characterised by one or more hyperparameters [2] . The posteriors of the hyperparameters are the main target for estimation and inference, and for present purposes are simply Poisson regression coefficients for three key variables: radiocarbon-dated count sequences of anthropogenic samples (a proxy for human activity); the taphonomic proxy data, which are also radiocarbon-dated count sequences; and probable sequences of oxygen isotopes from NGRIP ice cores that were also sampled in order to account for measurement and chronological uncertainty. After filtering the megafauna database in the ways suggested by Pelton and colleagues and constricting the temporal interval under consideration, we estimated REC model parameters with Markov chain Monte Carlo (MCMC) and then examined the posterior distributions. Regression models In order to make our extended analyses comparable to Broughton and Weitzel [3] , we followed their methods and calculated Spearman rank-order correlation coefficients for the newly filtered and temporally restricted data. The Spearman Rank-order Correlation Coefficient (denoted with the Greek letter ‘rho’) is a non-parametric statistic used to estimate the strength and direction of a monotonic relationship between two variables that can be rank-ordered (i.e., the data are at least ordinal). These correlations were estimated in R using standard built-in functions [11] . Positive values indicate a positive monotonic relationship between the relevant variables, and a negative value indicates an inverse relationship. The statistic ranges from –1 to +1 with the magnitude indicating the strength of the statistical association. We compared the Spearman correlation coefficients given the filtered/temporally-restricted data to those reported by Broughton and Weitzel. Reporting summary Further information on research design is available in the Nature Research Reporting Summary linked to this article.